FLOWERING LOCUS Tgenes control onion bulb formation and flowering Onion ( Allium cepa L.) is a biennial crop that in temperate regions is planted in the spring and, after a juvenile stage, forms a bulb in response to the lengthening photoperiod of late spring/summer. The bulb then overwinters and in the next season it flowers and sets seed. FLOWERING LOCUS T ( FT ) encodes a mobile signaling protein involved in regulating flowering, as well as other aspects of plant development. Here we show that in onions, different FT genes regulate flowering and bulb formation. Flowering is promoted by vernalization and correlates with the upregulation of AcFT2 , whereas bulb formation is regulated by two antagonistic FT- like genes. AcFT1 promotes bulb formation, while AcFT4 prevents AcFT1 upregulation and inhibits bulbing in transgenic onions. Long-day photoperiods lead to the downregulation of AcFT4 and the upregulation of AcFT1 , and this promotes bulbing. The observation that FT proteins can repress and promote different developmental transitions highlights the evolutionary versatility of FT. Onions are one of the oldest vegetables known to mankind and have been cultivated for more than 4,700 years. They are one of the most important vegetables, with 64 million tonnes of onions produced annually worldwide, exceeded only by tomatoes and cabbages [1] . Onion is a biennial plant, with the bulb being an overwintering stage of the life cycle, which, following a period of winter cold, flowers in the spring (a process known as vernalization) [1] . Vernalization has only been studied at the molecular level in a few species and, in all cases, results in the inhibition of a repressor, thereby allowing FLOWERING LOCUS T ( FT ) to be expressed [2] . FT has been shown to be the major component of the floral signal molecule, florigen [3] . Under inductive conditions, FT is produced in the phloem companion cells of the leaf and is transported to the apical meristem cells [4] , [5] , [6] where it forms a complex with 14-3-3 proteins and the bZIP transcription factor FD [7] , [8] , [9] , [10] , [11] . This complex, known as the florigen activation complex, is thought to translocate to the nucleus where it activates the floral meristem identity genes, thereby inducing flowering [12] . In Arabidopsis , vernalization results in the epigenetic silencing of the floral repressor FLC [13] . The silencing of FLC allows the photoperiodic induction of FT in the spring, which triggers flowering [3] . In sugar beet, vernalization involves two antagonistically acting FT genes [14] . Here FT1 inhibits the expression of FT2 , a gene that promotes flowering. After vernalization, FT1 is repressed allowing FT2 expression and flowering. In wheat and barley, vernalization also involves the regulation of a floral repressor [15] . In these plants, vernalization results in the upregulation of VRN1 (that encodes a protein similar to the Arabidopsis MADS box transcription factor proteins APETALA1 and FRUITFULL), which in turn downregulates the transcriptional repressor VRN2 , allowing FT expression and flowering [16] , [17] , [18] . In onion, vernalization is sufficient to induce flowering, although temperature and photoperiod influence the time taken for the inflorescence to appear [19] . Vernalization has not been studied at a molecular level in onion. Garner and Allard [20] , in 1920, first showed that onions develop bulbs in response to long-day (LD) photoperiods. Commercial onion varieties are classified as short, intermediate or LD length varieties, depending on the minimum daylength that induces bulbing, and provides an indication as to the latitude where a particular variety can be grown [1] . For example, LD onions are grown in temperate regions where bulbing is initiated once the daylength reaches at least 16 h per day, whereas short-day (SD) onions are grown in more tropical regions and require a daylength of only 12 h for bulbing [1] . This photoperiodic initiation of bulbing resembles the photoperiodic flowering in other plants [21] , [22] . As with flowering, daylength perception probably occurs in the leaves, while the response is in the meristem [1] , suggesting a mobile signal with properties similar to FT might be involved. In addition to regulating flowering, FT genes have been found to be involved in a range of physiological processes, suggesting that FT functions as a more general plant hormone. For example, in poplar an FT gene promotes vegetative growth and inhibition of bud set in response to warm temperatures and LD photoperiods [23] , [24] , [25] . In tomato and maize, in addition to promoting flowering, the FT genes ( SFT and ZCN8 , respectively) have been found to act as general regulators of growth [26] , [27] . A recent exciting discovery is that the potato FT orthologue StSP6A is involved in the SD induction of tuberization [28] . Here we show that FT genes play a key role in the controlling the major transitions in the biennial life cycle of onion: the photoperiodic induction of bulb formation and vernalization responsive flowering. Onion has at least six FT- like genes We set out to investigate whether FT -like genes are involved in controlling onion flowering and/or the photoperiodic induction of bulb formation. As the genome of onion has not been sequenced and there is only limited transcriptome data [29] , [30] , to identify FT -like transcripts, we performed GS-FLX sequencing of RNA isolated from the doubled haploid onion line CUDH2150. A BLAST search of our transcriptome data [31] identified six FT -like genes. Phylogenetic analysis of these, and other monocot FT proteins, revealed that all six FT-like proteins belonged to the FT-like group ( Fig. 1a and Supplementary Fig. S1 ). Previous work defined two groups of FT-like proteins, I and II [32] , and our work suggests that both these groups can be further divided to make four subgroups: FT-like IA, IB, IIA and IIB ( Fig. 1a ). Subgroup IA contains AcFT1 and AcFT2 as well as the monocot FTs implicated in regulating flowering in rice [33] (Hd3a and RFT1), barley [34] , [35] (HvFT1 and HvFT2) and orchid [36] (CgFT; Fig. 1a , proteins marked with asterisk). AcFT4 is positioned within subgroup IIA that also contains the FT-like proteins associated with the flowering of maize [32] (ZmZCN8) and barley [34] , [35] (HvFT3). AcFT3, AcFT5 and AcFT6 proteins are located in FT-like subgroup IB and a role has not been established for any of the proteins within this subgroup. 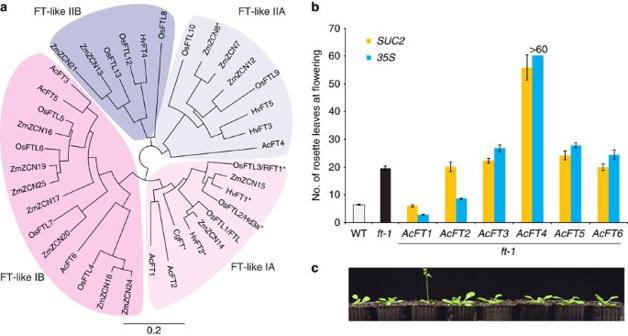Figure 1: Onion has at least sixFT-like genes that have differing activities in transgenicArabidopsis. (a) Phylogram of FT-like protein sequences from different monocot plants. Four subgroups are indicated. The sequences are from onion (Allium cepa, Ac), rice (Oryza sativa, Os), maize (Zea mays, Zm), barley (Hordeum vulgare, Hv) and spring orchid (Cymbidium goeringii, Cg). FTs with asterisks have been shown to promote flowering. SeeSupplementary Fig. S1for full protein alignment and Genbank accession details. (b) Complementation of theArabidopsis ft-1 mutant with onionFT-like genes expressed under the constitutive 35S promoter (blue) or phloem-specificSUC2promoter (yellow). Flowering time as determined by number of rosette leaves at flowering of representative lines grown in LD. Note: 6 out of 1635S:AcFT4plants did not flower, while the remaining plants flowered with more than 33 leaves. Data represent a minimum of 10 plants scored for each line ±s.e.m. (c) Photo of35S:AcFTlines grown in LD, withAcFT1flowering and floral buds visible on WT and35S:AcFT2plants (plants are in the same order as the panelbgraph). Figure 1: Onion has at least six FT -like genes that have differing activities in transgenic Arabidopsis . ( a ) Phylogram of FT-like protein sequences from different monocot plants. Four subgroups are indicated. The sequences are from onion ( Allium cepa , Ac), rice ( Oryza sativa , Os), maize ( Zea mays , Zm), barley ( Hordeum vulgare , Hv) and spring orchid ( Cymbidium goeringii , Cg). FTs with asterisks have been shown to promote flowering. See Supplementary Fig. S1 for full protein alignment and Genbank accession details. ( b ) Complementation of the Arabidopsis ft -1 mutant with onion FT -like genes expressed under the constitutive 35S promoter (blue) or phloem-specific SUC2 promoter (yellow). Flowering time as determined by number of rosette leaves at flowering of representative lines grown in LD. Note: 6 out of 16 35S:AcFT4 plants did not flower, while the remaining plants flowered with more than 33 leaves. Data represent a minimum of 10 plants scored for each line ±s.e.m. ( c ) Photo of 35S:AcFT lines grown in LD, with AcFT1 flowering and floral buds visible on WT and 35S : AcFT2 plants (plants are in the same order as the panel b graph). Full size image Next, we tested the ability of the onion FT -like genes to complement the late flowering Arabidopsis ft -1 mutant. Transgenic Arabidopsis ft -1 plants expressing each of the six FT -like complementary DNA under the control of the strong constitutive cauliflower mosaic virus 35S promoter were produced and their flowering time analysed ( Fig. 1b and Supplementary Fig. S2 ). 35S:AcFT1 flowered significantly earlier than wild type and 35S:AcFT2 slightly later than wild type, but significantly earlier than the ft -1 mutant. Thus, both AcFT1 and AcFT2 encode proteins that are capable of functioning to promote flowering. In contrast, 35S:AcFT4 plants were very late flowering, with the majority of plants remaining vegetative after producing over 60 leaves ( Fig. 1b ). The 35S:AcFT3 , 35S:AcFT5 and 35S:AcFT6 constructs were unable to complement the ft -1 mutant. The 35S promoter results in expression throughout the plant, including the apical meristem cells where the floral transition occurs. To examine whether the onion FT -like proteins are capable of acting as a mobile floral signal in Arabidopsis , we expressed the six FT -like cDNAs under the control of the phloem-specific promoter, SUC2 . Consistent with the 35S promoter results, SUC2 -expressed AcFT3 , AcFT5 and AcFT6 did not complement ft-1 . The SUC2:AcFT1 plants flowered early, indicating that AcFT1 can function as a mobile signal molecule. Interestingly, in contrast to 35S:AcFT2 that partially complements the Arabidopsis ft -1 mutant, most of the SUC2:AcFT2 plants did not have altered flowering time ( Fig. 1b and Supplementary Fig. S3 ), suggesting that AcFT2 has limited ability to act as a mobile signal. The SUC2:AcFT4 plants flowered significantly later than ft -1. Consistent with AcFT4 acting as a mobile inhibitor of flowering by antagonizing FT function in the apex, the endogenous Arabidopsis FT genes ( FT and TSF ) are still expressed in the leaves; however, floral meristem identity genes are not upregulated in the apex ( Supplementary Fig. S4 ). AcFT2 expression correlates with flowering Previous work has shown that vernalization is sufficient to induce flowering in onion [19] . Consistent with this, we have found that flowering is induced in onion bulbs stored in the cold (4 °C) and dark for 3–4 months ( Supplementary Fig. S5 ), indicating that a photoperiodic signal is not necessary to induce onion flowering in the spring. To discover whether any of the onion FT -like genes are potentially involved in regulating flowering, we examined the expression of the FT -like genes at various stages throughout development and in plants grown in SD and LD photoperiods ( Supplementary Fig. S6 ). Only the expression of AcFT2 correlated with flowering, implicating this gene as encoding a key floral signal molecule. The expression of AcFT2 was either not detected or at very low levels in seedlings and older plants before or after bulb formation ( Fig. 2 ). However, AcFT2 is expressed at high levels in leaves of flowering bulbs grown in either SD or LDs ( Fig. 2 ). Next, we examined the expression of the FTs in vernalized and non-vernalized onion bulbs stored in the dark. While before vernalization AcFT2 is not expressed in the bulb, after vernalization AcFT2 is expressed at high levels in the central bud tissue that will form the floral inflorescence ( Fig. 2 ). AcFT1 is not expressed in the vernalized bulb tissue ( Supplementary Fig. S5 ). These results indicate that AcFT2 is a strong candidate for the key regulator of flowering in onion. 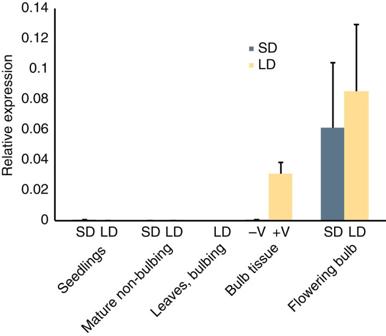Figure 2:AcFT2expression correlates with flowering. Expression ofAcFT2in leaf tissue from seedlings with 3–4 leaves (young), plants with ~10 leaves before bulb formation (mature), and bulbing plants (bulbing) and central bud tissue from bulbs (bulb tissue) non-vernalized (−V) or vernalized in the dark for 3 months (+V), leaves from flowering plants (flowering bulb). Samples were taken from plants grown at 20 °C under SD (8 h light: 16 h dark) and LD (16 h light: 8 h dark) photoperiods (except bulbing plants, as bulbs do not form in SD). Data represent an average ±s.e.m. of three biological replicates, with transcripts normalized toβ-tubulin. Figure 2: AcFT2 expression correlates with flowering. Expression of AcFT2 in leaf tissue from seedlings with 3–4 leaves (young), plants with ~10 leaves before bulb formation (mature), and bulbing plants (bulbing) and central bud tissue from bulbs (bulb tissue) non-vernalized (−V) or vernalized in the dark for 3 months (+V), leaves from flowering plants (flowering bulb). Samples were taken from plants grown at 20 °C under SD (8 h light: 16 h dark) and LD (16 h light: 8 h dark) photoperiods (except bulbing plants, as bulbs do not form in SD). Data represent an average ±s.e.m. of three biological replicates, with transcripts normalized to β-tubulin . Full size image AcFT1 and AcFT4 expression suggests they control bulbing In onion, seedlings need reach a certain developmental stage before they form bulbs. Bulb formation then only occurs when under inductive photoperiods. In our growth conditions, onion cultivar CUDH2107 did not form bulbs when grown under a SD photoperiod (8 h light: 16 h dark), but did bulb in LD photoperiod (16 h light: 8 h light). To investigate the role of the FT -like genes in bulb formation, we first examined the FT genes at the following three key stages of development: seedlings, mature non-bulbing plants and flowering bulbs, in both SD and LD photoperiods ( Fig. 3a ). The expression of AcFT3 , AcFT5 and AcFT6 (the FT -like genes in subgroup IB) were similar at the three stages of development and did not appear to be strongly affected by daylength ( Supplementary Fig. S7 ). However, the expression of AcFT1 and AcFT4 were influenced by developmental stage and photoperiod ( Fig. 3 ). In leaves of young seedlings, AcFT1 is expressed at very low levels, while AcFT4 is expressed at relatively high levels in both SD and LD photoperiods ( Fig. 3a ). In leaves from plants competent to initiate bulb formation (but lacking visible bulbs), AcFT1 is only expressed in LD grown plants (that will form bulbs) but is not expressed in SD grown plants (that will not form bulbs). AcFT4 had the opposite expression pattern that is, it was only detected in SD grown plants ( Fig. 3a ). A similar pattern of AcFT1 and AcFT4 expression was observed when bulbs produced in the previous season were grown in SD and LD photoperiods ( Fig. 3a ). These results suggest a model where the LD induction of bulbing involves the downregulation of AcFT4 and the upregulation of AcFT1 . This model is consistent with the complementation experiments ( Fig. 1 ) where AcFT4 acts as an inhibitor and AcFT1 acts as a promoter of Arabidopsis flowering. In young seedlings, premature bulbing would be prevented by the expression of AcFT4 and the lack of AcFT1 . 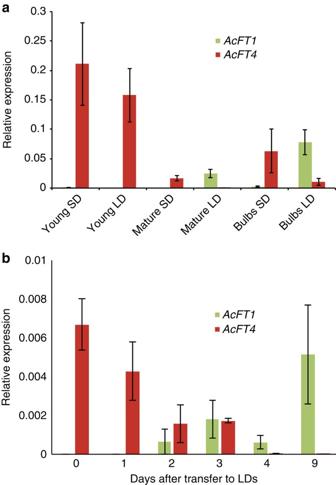Figure 3:AcFT1is induced andAcFT4is repressed by conditions that induce bulb formation. (a) Expression ofAcFT1andAcFT4in leaf tissue from young plants with 3–4 leaves (young), plants with ~10 leaves before bulb formation (mature) and bulbs from previous season grown to have 4–5 fully expanded leaves (bulbs). (b) Expression ofAcFT1andAcFT4after transfer from SD to LD. Mature onion seedlings were grown under SD for 14 weeks and then transferred to LD. Leaf samples were taken at ZT5. All plants were grown at 20 °C under SD (8 h light: 16 h dark) or LD (16 h light: 8 h dark) photoperiods. The data represent an average ±s.e.m. of three individual plants, with transcripts normalized toβ-tubulin. Figure 3: AcFT1 is induced and AcFT4 is repressed by conditions that induce bulb formation. ( a ) Expression of AcFT1 and AcFT4 in leaf tissue from young plants with 3–4 leaves (young), plants with ~10 leaves before bulb formation (mature) and bulbs from previous season grown to have 4–5 fully expanded leaves (bulbs). ( b ) Expression of AcFT1 and AcFT4 after transfer from SD to LD. Mature onion seedlings were grown under SD for 14 weeks and then transferred to LD. Leaf samples were taken at ZT5. All plants were grown at 20 °C under SD (8 h light: 16 h dark) or LD (16 h light: 8 h dark) photoperiods. The data represent an average ±s.e.m. of three individual plants, with transcripts normalized to β-tubulin . Full size image In Arabidopsis and other plants, FT is rapidly upregulated when plants are shifted from non-inductive conditions to an inductive photoperiod [4] , [37] . To investigate the timescale of the photoperiodic regulation of AcFT1 and AcFT4 , plants were shifted from SD to LD photoperiod. All the onion plants shifted into LD formed bulbs, while the onions that remained in SD did not. AcFT4 expression was reduced after just 1 day in LDs and almost no expression was observed after 4 days ( Fig. 3b ). AcFT1 showed the opposite pattern of expression, with AcFT1 expression being detected after 2 days in LDs ( Fig. 3b ). Thus, the FT -like genes rapidly respond to photoperiod, consistent with them playing a key role in the photoperiodic induction of bulbing. In summary, our data indicate that AcFT4 and AcFT1 are key regulators of bulb formation, with AcFT4 functioning as an inhibitor of bulbing and AcFT1 as a promotor of bulbing. AcFT1 and AcFT4 control bulb formation in transgenic onions To further investigate the role of the FT -like genes, we set out to generate transgenic onion plants overexpressing the genes implicated in bulb formation ( AcFT1 and AcFT4 ) and flowering ( AcFT2 ). The onion transformation protocol is technically demanding with low transformation efficiency. Fortunately, we were able to recover a few AcFT1 and AcFT4 transformants. Overexpression of the AcFT1 cDNA using a 35S promoter resulted in a dramatic phenotype, with bulb-like structures being formed while still in tissue culture ( Fig. 4a ), compared with the normal vegetative development of the 35S:AcFT4 plants ( Fig. 4b ). These structures had increased expression of sucrose:sucrose 1-fructosyltransferase ( 1-SST ; Fig. 4c ), a gene that is normally upregulated on bulbing [38] , providing further evidence that AcFT1 promotes bulb formation. In contrast, overexpression of AcFT4 had a similar phenotype to the control plants before bulbing. However, while the control plants produced bulbs in late spring, the 35S:AcFT4 plants did not ( Fig. 4d,e ). The 35S:AcFT4 plants continued growing vegetatively into winter, while the leaves of control plants died back in the autumn leaving only bulbs ( Supplementary Fig. S8 ). Next, we analysed the expression of the FT -like genes in the transgenic 35S:AcFT4 plants and controls. As expected, the bulbing control plants had very low levels of AcFT4 and relatively high levels of AcFT1 ( Fig. 4f ). In contrast, in the transgenic plants overexpressing AcFT4 , AcFT1 expression was strongly inhibited ( Fig. 4f ). 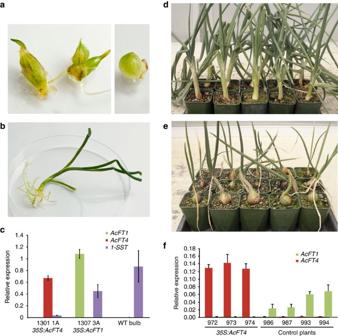Figure 4: Overexpression ofAcFT4prevents bulbing and inhibits expression ofAcFT1. (a)35S:AcFT1plants form bulb-like structures in tissue culture (independent lines are shown in separate photographs) and in comparison (b)35S:AcFT4plants that are the same age, show normal vegetative growth in tissue culture. (c) Relative expression ofAcFT1, AcFT2and the bulb marker1-SSTin representative35S:AcFT41and35S:AcFT4lines grown in tissue culture and bulb tissue from a mature wild-type plant. (d)35S:AcFT4plants and (e) control plants (derived from calli generated in same experiment as35S:AcFT4plants but not expressingGFPorAcFT4) grown in glasshouse conditions and photographed in late summer (28 Feb 2013). Note: the 35S:AcFT4plants shown indwere derived from the same transgenic callus and are therefore are probably from a single transgenic event. (f) Expression ofAcFT4andAcFT1in representative35S:AcFT4and control plants. The expression data represent an average ±s.e.m. of three individual plants, with transcripts normalized toβ-tubulin. Figure 4: Overexpression of AcFT4 prevents bulbing and inhibits expression of AcFT1 . ( a ) 35S:AcFT1 plants form bulb-like structures in tissue culture (independent lines are shown in separate photographs) and in comparison ( b ) 35S:AcFT4 plants that are the same age, show normal vegetative growth in tissue culture. ( c ) Relative expression of AcFT1, AcFT2 and the bulb marker 1-SST in representative 35S:AcFT41 and 35S:AcFT4 lines grown in tissue culture and bulb tissue from a mature wild-type plant. ( d ) 35S : AcFT4 plants and ( e ) control plants (derived from calli generated in same experiment as 35S:AcFT4 plants but not expressing GFP or AcFT4 ) grown in glasshouse conditions and photographed in late summer (28 Feb 2013). Note: the 35S: AcFT4 plants shown in d were derived from the same transgenic callus and are therefore are probably from a single transgenic event. ( f ) Expression of AcFT4 and AcFT1 in representative 35S:AcFT4 and control plants. The expression data represent an average ±s.e.m. of three individual plants, with transcripts normalized to β-tubulin . Full size image Together, these results are consistent with the expression data presented in Fig. 3 and indicates that under LD photoperiods the downregulation of AcFT4 allows AcFT1 upregulation to occur, which then triggers bulb formation. Structural changes in FTs underlie differences in function Our results indicate that there are three FT-like proteins that have different roles in onion development. Although AcFT1 and AcFT2 share ~83% amino-acid similarity, AcFT1 promotes bulbing, while AcFT2 regulates flowering. The sequence variation between the two proteins results in functional differences when overexpressed in Arabidopsis , with AcFT2 having a reduced ability to ectopically upregulate FT targets in the leaves ( Supplementary Fig. S9 ) and act as a mobile signal ( Fig. 1b and Supplementary Fig. S2 ). The different properties of AcFT1 and AcFT2, together with their different patterns of expression, probably determine their abilities to perform distinct functions inducing bulbing and flowering, respectively. We therefore set out to examine the structural differences between the different AcFT proteins. FT proteins interact with the bZIP DNA-binding protein FD via a 14-3-3 protein to make what is known as a florigen activation complex [11] . Therefore, the different activities of the onion FT proteins might be due to their affinity for the 14-3-3 protein. AcFT2 differs from AcFT1 at a number of residues ( Supplementary Fig. S1 ). Analysis of the position of these differences within the FT structure from rice (Hd3a) [11] revealed that non-conservative changes in key residues within the FT/14-3-3 interface are likely to alter interaction with 14-3-3 proteins. This suggests that AcFT1 and AcFT2 interact with different 14-3-3 proteins ( Fig. 5a,b ). Even more striking, residue changes within AcFT4 (the FT that inhibits bulbing) are predicted to completely disrupt the interface with 14-3-3 ( Fig. 5c ), suggesting AcFT4 either interacts with another protein or functions as a dominant-negative protein. 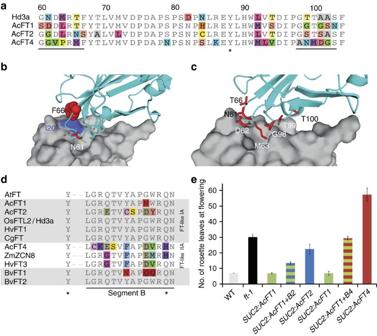Figure 5: Structural and functional analysis of the onionFT-like proteins. (a) Partial amino-acid alignment between rice Hd3a and AcFT1, AcFT2 and AcFT4 showing non-conserved residues, with those located at the interface between FT and 14-3-3 underlined. (b) Structure of Hd3a (cyan) bound to 14-3-3 protein (grey) showing the positions of the residues that are not conserved in AcFT2 (red). The residue at the equivalent position to Hd3a phenylalanine 66 (F66) (red) is a serine in AcFT2, which is predicted to disrupt the packing to residue isoleucine 204 (I204) (blue) in 14-3-3. (c) The non-conserved residues in AcFT4, that are predicted to disrupt the interaction between Hd3a (cyan) and 14-3-3 protein (gray), are highlighted in red. (d) Partial amino-acid alignment of FT sequences fromArabidopsis(Arabidopsis thaliana, At), onion (Allium cepa, Ac), rice (Oryza sativa, Os), barley (Hordeum vulgare, Hv), maize (Zea mays, Zm), spring orchid (Cymbidium goeringii, Cg) and sugar beet (Beta vulgaris, Bv). Asterisks on the bottom row indicate Tyr-85 (Y)/His-88 (H) and Gln-140 (Q)/Asp-144 (D) residues distinguishing FT-like and TFL1-like members. The black bar indicates the conserved segmental region B, corresponding to the external loop of FT. (e) Complementation of theArabidopsis ft-1 mutant with AcFT1, AcFT2 and AcFT4 and chimeric constructs in which segment B from AcFT1 was replaced with segment B from AcFT2 (AcFT1+B2) or AcFT4 (AcFT1+B4). All constructs were expressed under the phloem-specificSUC2promoter. Flowering time as determined by number of rosette leaves at flowering of representative lines grown in LD. Data represent a minimum of 10 plants scored for each line ±s.e.m. Figure 5: Structural and functional analysis of the onion FT -like proteins. ( a ) Partial amino-acid alignment between rice Hd3a and AcFT1, AcFT2 and AcFT4 showing non-conserved residues, with those located at the interface between FT and 14-3-3 underlined. ( b ) Structure of Hd3a (cyan) bound to 14-3-3 protein (grey) showing the positions of the residues that are not conserved in AcFT2 (red). The residue at the equivalent position to Hd3a phenylalanine 66 (F66) (red) is a serine in AcFT2, which is predicted to disrupt the packing to residue isoleucine 204 (I204) (blue) in 14-3-3. ( c ) The non-conserved residues in AcFT4, that are predicted to disrupt the interaction between Hd3a (cyan) and 14-3-3 protein (gray), are highlighted in red. ( d ) Partial amino-acid alignment of FT sequences from Arabidopsis ( Arabidopsis thaliana , At), onion ( Allium cepa , Ac), rice ( Oryza sativa , Os), barley ( Hordeum vulgare , Hv), maize ( Zea mays , Zm), spring orchid ( Cymbidium goeringii , Cg) and sugar beet ( Beta vulgaris , Bv). Asterisks on the bottom row indicate Tyr-85 (Y)/His-88 (H) and Gln-140 (Q)/Asp-144 (D) residues distinguishing FT-like and TFL1-like members. The black bar indicates the conserved segmental region B, corresponding to the external loop of FT. ( e ) Complementation of the Arabidopsis ft -1 mutant with AcFT1, AcFT2 and AcFT4 and chimeric constructs in which segment B from AcFT1 was replaced with segment B from AcFT2 (AcFT1+B2) or AcFT4 (AcFT1+B4). All constructs were expressed under the phloem-specific SUC2 promoter. Flowering time as determined by number of rosette leaves at flowering of representative lines grown in LD. Data represent a minimum of 10 plants scored for each line ±s.e.m. Full size image Two regions of FT are critical for the promotion of flowering, segment B (a surface-exposed loop region) and the residue Y85, and are the key functional differences between FT and the floral repressor TFL1. Replacement of the segment B residues of FT, with those from TFL1, confers the repressive ability on the chimeric protein [39] , [40] . Similarly, the repressive function of the sugar beet FT, BvFT1, is explained by sequence differences in B [14] . Examination of this region of the AcFT proteins revealed differences, with both AcFT2 and AcFT4 having sequences not found in other FTs ( Fig. 5d ). To test the functional implications of these differences, we transformed Arabidopsis ft-1 mutants with constructs in which AcFT1 contained the segment B sequences from either AcFT2 or AcFT4 (referred to as AcFT1+B2 and AcFT1+B4 , respectively). Introducing segment B from AcFT2 into AcFT1 (that is, construct AcFT1+B2 ) reduced its ability (activity and/or mobility) to promote Arabidopsis flowering, although the resulting transformants were not as late as the SUC2:AcFT2 controls indicating that differences at other residues also contribute to the differences between the two proteins ( Fig. 5e and Supplementary Fig. S10 ). Introducing segment B from AcFT4 into AcFT1 (that is, construct AcFT1+B4 ) abolished its ability to promote flowering. However, unlike SUC2:AcFT4 , this construct did not repress flowering ( Fig. 5e and Supplementary Fig. S10 ). Overall, the structural and functional studies support the idea that AcFT1 , AcFT2 and AcFT4 have evolved specialist roles to control the key developmental transitions in onion. It was 93 years ago that Garner and Allard [20] first demonstrated that onion bulbing is induced by LD photoperiods. While physiological experiments have revealed the importance of plant age, light quality and photoperiod for the induction of bulb formation [21] , [41] , [42] , [43] , the ‘hormone’ controlling this process has not been identified. Here we provide evidence that genes encoding FT-like proteins play a key role in controlling both onion bulb formation and flowering. A model of the roles of FT -like genes in the seasonal control of onion development is presented in Fig. 6 . Our evidence indicates that in juvenile plants and those grown under non-inductive photoperiod, AcFT4 functions to prevent the upregulation of AcFT1 . Once the plants are mature and daylength reaches a critical length, AcFT4 is downregulated and AcFT1 is upregulated leading to the initiation of bulb formation. Consistent with this model, constitutive expression of AcFT4 prevents both AcFT1 upregulation and bulb formation. A similar regulatory pathway has evolved in sugar beet, where two FT s with opposite expression profiles and antagonistic functions control flowering [14] , [44] . Here the related FT s, BvFT1 and BvFT2 are expressed in the leaves of vegetative and reproductive plants, respectively. BvFT1 functions as a floral inhibitor by repressing BvFT2 . Under inductive conditions (after vernalization and in LD photoperiod), BvFT1 is downregulated, thereby allowing BvFT2 to be expressed and flowering to occur. The inhibitory activity of BvFT1 is the result of specific amino-acid changes within segment B [14] . Similar to BvFT1 , the antagonistic function of AcFT4 is evident in Arabidopsis where its overexpression results in a significant delay in flowering. To investigate whether segment B is responsible for the inhibitory activity of AcFT4, segment B of AcFT1 (a strong promoter of Arabidopsis flowering) was replaced with AcFT4 sequences ( Fig. 5d ). While this construct was no longer able to promote flowering, it did not repress flowering ( Fig. 5e ), indicating other sequence differences are involved. Interestingly, AcFT4 also has a number of amino-acid changes that are predicted to prevent its interaction with the 14-3-3 protein that mediates the interaction between FT and FD [11] ( Fig. 5c ). Further work will be needed to understand the inhibitory activity of AcFT4 and whether, for example, it acts as a transcriptional repressor of FT targets (as is the case for TFL1 (refs 45 , 46 )) or by competing with FT as a dominant negative [47] . 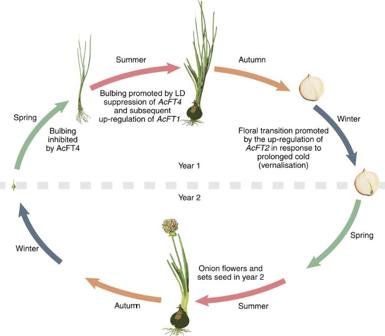Figure 6: Model of the role of theFT-like genes in onion. An onion seedling that is planted in the spring (left) is initially prevented from forming a bulb by the expression ofAcFT4. Once the onion plant is mature and the daylength has reached a critical length,AcFT4is downregulated allowing the upregulation ofAcFT1, which induces bulb formation. The onion plant then overwinters as a bulb and during this time, the upregulation ofAcFT2in response to prolonged cold results in the induction of flowering (a process known as vernalization). The onion plant then flowers and sets seed during the spring/summer of its second year of growth. Figure 6: Model of the role of the FT -like genes in onion. An onion seedling that is planted in the spring (left) is initially prevented from forming a bulb by the expression of AcFT4 . Once the onion plant is mature and the daylength has reached a critical length, AcFT4 is downregulated allowing the upregulation of AcFT1 , which induces bulb formation. The onion plant then overwinters as a bulb and during this time, the upregulation of AcFT2 in response to prolonged cold results in the induction of flowering (a process known as vernalization). The onion plant then flowers and sets seed during the spring/summer of its second year of growth. Full size image In our model, we propose that AcFT1 promotes bulb formation, while AcFT2 promotes flowering. Our phylogenic analysis ( Fig. 1a ) suggests that the two FT genes (which share 83% amino-acid similarity) may have evolved through gene duplication and neofunctionalization. Other plants where related FT genes have evolved distinct roles include potato, where two FTs (StSP3D and StSP6A) appear to encode mobile signals that promote flowering and tuberization, respectively [28] , and poplar where FT2 is expressed during vegetative growth and likely regulates growth cessation and bud set, while FT1 is predominantly expressed in late winter and is involved in floral induction (although FT2 might also play a role) [23] , [25] , [44] . How might FTs have evolved different roles? The ability of FT to induce flowering requires the presence of FT protein within the apical meristem and for FT to interact with components of the floral activating complex (a 14-3-3 protein and FD) to activate floral meristem identity genes, such as LFY and AP1 (refs 7 , 8 , 9 , 10 , 11 ). While we predict that AcFT2 induces flowering by activating floral meristem identity genes, the induction of bulb formation by AcFT1 will involve different and unknown targets. Our studies in Arabidopsis revealed that AcFT1 and AcFT2 have differing abilities to complement the ft-1 mutant and indicate that the functional specificity of the two FTs might, at least in part, be due to differences in their sequence. Swapping segment B from AcFT2 into AcFT1 revealed that sequences both within this region and within the rest of the protein are responsible for the differing ability of the two FTs to complement the Arabidopsis ft-1 mutant. For example, key amino-acid differences within the 14-3-3 interaction interface are predicted to influence the ability of the AcFT1 to bind other proteins and might result in the preferential binding to a different 14-3-3 protein and therefore form a different complex. Differences in the expression and movement of AcFT1 and AcFT2 are also likely to be key to the functional specificity of the two FTs. The photoperiodic induction of AcFT1 occurs in the leaves ( Fig. 3 ) and AcFT1 protein is probably transported to the vegetative meristematic cells where it induces bulb formation. Consistent with AcFT1 acting as a mobile signal, SUC2:AcFT1 fully complemented the Arabidopsis ft-1 mutant ( Fig. 1b ). In contrast, AcFT2 is expressed in the bulb meristematic tissue after vernalization ( Fig. 2 ). It is therefore possible that AcFT2 is expressed within the tissues it acts in and might not need to (or be able to) be transported. Consistent with this idea, while constitutive expression of AcFT2 promoted Arabidopsis flowering, AcFT2 had limited floral inductive activity when expressed in the phloem companion cells (using the SUC2 promoter; Fig. 1b ). AcFT2 is also expressed in the leaves of onion plants that are flowering ( Fig. 2 ). A feature of the vernalization response is that plants retain an epigenetic memory of the cold that is passed on through cell division. Thus, one explanation for the leaf expression of AcFT2 is that once it is upregulated in the meristematic cells, it remains turned on in leaves originating from these cells. Future work using additional transgenic onion lines will be needed to unequivocally demonstrate the roles of the different FT genes and to understand the molecular basis of their specific roles in flowering and bulb formation. The discovery that bulb formation is induced by the downregulation of AcFT4 and the upregulation of AcFT1 in response to LD photoperiods provides the molecular tools to investigate the difference between SD-, intermediate- and LD onion varieties (note: unlike SD flowering that requires days to be shorter than a critical length for flowering, all onions bulb when the daylength is longer than a critical length). Molecular genetic analysis in a wide range of plants has revealed that sequence changes in components of the circadian clock [48] , [49] , [50] , [51] and downstream components [51] , including FT genes [52] , [53] , underlie the variation in daylength required to induce flowering. It is therefore likely that the adaptation of onions to bulb at the appropriate time in different latitudes involves similar mechanisms. Leek is an important Allium crop that does not form bulbs and therefore lacks a photoperiodic requirement. These features allow leaks to be planted throughout the season and grown over a wide range of latitudes [1] . Interestingly, the 35S:AcFT4 plants that do not bulb have a similar appearance to leeks and continued growing vegetatively into the winter without their foliage dying off ( Fig. 4 ; Supplementary Fig. S8 ). This suggests that the large phenotypic differences between onion and leek might be due to a simple genetic change. While the presence of large bulbs is a distinct feature of onions, most members of the Allium genus form some type of storage organ. For example, garlic cloves (the storage organ) are formed from swollen bladeless inner sheaths, but unlike in onion no storage occurs in foliage leaf bases, whereas chive storage is in foliage leaf bases (but bulbs are absent) [1] . It will be interesting to discover the role FT -like genes play in other Alliums , and whether genetic variation within FT genes, or their targets explains their phenotypic variation. In summary, this work provides the first evidence that FT genes control both floral induction and bulb formation in onion. It also adds to the growing body of evidence that FT genes not only regulate flowering, but play a wider role in controlling developmental decisions. Plant materials Doubled haploid onion lines CUDH2150 and CUDH2107 were obtained from the Cornell University [54] . Seed lots were sown in spring either directly as seed or as transplants in Jiffy 7 plug (Jiffy Corp) and grown in Black Magic seed-raising mix (Yates Orica, New Zealand). Onion and Arabidopsis plants were grown under either LD (16 h light: 8 h dark) or SD (8 h light: 16 h dark) photoperiod in plant growth rooms maintained at 20 °C with 30–40% humidity and a light intensity of ~115 μmol m −2 s −1 . Identification and cloning of onion FT -like genes Onion FT -like sequences were identified from our transcriptome data deposited at NCBI BioProject 60277 (ref. 31 ) using TBLASTN. Full-length cDNA sequences were obtained from six partial FT -like sequences ( AcFT1-6 ) using the Invitrogen GeneRacer RNA ligase-mediated rapid amplification of 5′ and 3′ cDNA ends (RLM-RACE) kit and these have been deposited in GenBank Nucleotide core database under accession codes KC485348-53 . Full-length PCR products of each FT were cloned from ‘CUDH2150’ using pCR8/GW/TOPO TA Cloning Kit (Invitrogen). Correct orientation was confirmed by sequencing. The TOPO-based clones were then linearized with either Xba I or Xho I, and recombined into pB2GW7 with LR Clonase (Invitrogen), thereby producing a binary vector containing CaMV 35S: AcFT . To construct the SUC2 promoter-driven constructs, first the 35S promoter in pB2GW7 was replaced with the SUC2 promoter from pAF12 (ref. 55 ). pB2GW7 was digested with Sac I/ Eco RI to release the 35S promoter. The att RI site was lost in this reaction, so it was replaced with a PCR fragment that contained Sac I– Xba I sites at the 5′-end and an Eco RI site at the 3′-end. Ligated together, Sac I/ Eco RI, this reforms pB2GW7 without the 35S promoter. The SUC2 promoter was PCR amplified from the pAF12 vector, with Sac I and Xba I sites on the 5′- and 3′-ends respectively, and cloned into the promoterless pB2GW7 vector at these sites. Plant transformation SUC2:AcFT and 35S:AcFT binary vectors were transformed into Agrobacterium tumefaciens GV3101 by electroporation. Arabidopsis were transformed using the method of Martinez-Trujillo et al. [56] as follows: Agrobacterium harbouring the binary vector were streaked onto LB media plates with selective antibiotics and incubated at 28 °C for 2 days. The bacteria were then scraped off the plate and resuspended in 10 ml of infiltration media (0.5 × MS (Duchefa), 0.05% Silwett L-77 (Lehle Seeds), 5% sucrose) to an OD 600 ~2 and droplets of this solution were pipetted onto unopened flower buds of Arabidopsis thaliana ft-1 mutants [56] . This was repeated three times in 2–3-day intervals. The resulting seed was sown on seed-raising mix and transformants selected by spraying the young seedlings with Basta herbicide (glufosinate ammonium; Bayer) at 120 mg l −1 . Onions were transformed with a binary vector containing the AcFT1 or AcFT4 cDNA under the control of the 35S promoter, along with the eGFP-ER reporter gene and the Bar selectable marker-, using the method of Eady et al. [57] as follows: immature embryos from onion seeds (‘Pukekohe LongKeeper’) incubated overnight at 4 °C were isolated and cut into ~1 mm lengths before transfer into 50 μl liquid P5 medium. Agrobacterium , resuspended in 0.4 ml liquid P5 to an OD 550 of 0.4–0.6, was added and embryos were vortexed for 30 s, and then placed under vacuum (~20 in Hg) for 30 min before blot drying on filter paper and transferred to P5 medium solidified with 0.4% Phytagel (Gellan Gum). After 6 days cocultivation, embryo pieces were transferred to P5 plus 2.5 mg l −1 phosphinothricin and 200 mg l −1 timentin. These embryo pieces were cultured in the dark under the same conditions as described for the production of secondary embryos [58] . Cultures were transferred to fresh medium every 2 weeks. After three to four transfers, growing material was transferred to P5 plus 5 mg l −1 phosphinothricin and grown for a further 8 weeks. During this time, pieces of putative transgenic tissue that reached ~2 mm 2 were transferred to regeneration medium [58] . Shoot cultures were maintained for 12 weeks and developing shoots were transferred to ½ MS medium plus 20 mg l −1 geneticin to induce rooting. Rooted plants were either transferred to ½ MS plus 120 g l −1 sucrose to induce bulb formation or to soil in the glasshouse (12 h 12–23 °C day, 12 h 4–16 °C night). Expression of the transgenes were confirmed by reverse transcriptase–PCR using primers given in Supplementary Table S1 . Analysis of gene expression Plant tissue was harvested into liquid nitrogen. Total RNA was extracted using the Invitrogen Plant RNA Purification Reagent, according to the manufacturer's instructions, but with an addition 30 min incubation in the reagent for onion tissue. RNA concentrations were determined using a NanoDrop 8000 (ThermoScientific). Reverse transcription was carried out with 1 μg of total RNA in 20 μl volumes using Invitrogen SuperScriptIII according to the manufacturer’s instructions. First-strand cDNA was diluted 30-fold, and 3 μl of this was used in each 10 μl reaction. Real-time PCR was performed using the Roche LC480 machine and Light-Cycler 480 SYBR Green I Master mix (Roche). Relative gene expression levels were calculated using the 2(2delta delta C(T)) method using Roche LC480 software. β-tubulin was used as the reference gene. Primers used for quantitative reverse transcriptase–PCR experiments can be found in Supplementary Table S1 . Accession codes: Sequence of AcFT1-6 cDNAs have been deposited in GenBank Nucleotide core database under accession codes KC485348 to KC485353 . How to cite this article: Lee, R. et al. FLOWERING LOCUS T genes control onion bulb formation and flowering. Nat. Commun. 4:2884 doi: 10.1038/ncomms3884 (2013).